Codon-reading specificities of mitochondrial release factors and translation termination at non-standard stop codons A key feature of mitochondrial translation is the reduced number of transfer RNAs and reassignment of codons. For human mitochondria, a major unresolved problem is how the set of stop codons are decoded by the release factors mtRF1a and mtRF1. Here we present three-dimensional structural models of human mtRF1a and mtRF1 based on their homology to bacterial RF1 in the codon recognition domain, and the strong conservation between mitochondrial and bacterial ribosomal RNA in the decoding region. Sequence changes in the less homologous mtRF1 appear to be correlated with specific features of the mitochondrial rRNA. Extensive computer simulations of the complexes with the ribosomal decoding site show that both mitochondrial factors have similar specificities and that neither reads the putative vertebrate stop codons AGA and AGG. Instead, we present a structural model for a mechanism by which the ICT1 protein causes termination by sensing the presence of these codons in the A-site of stalled ribosomes. The mitochondrion is an organelle found in most eukaryotic cells with critical functions for ATP production. Although the mitochondrion has its own DNA and translation system [1] , the human mitochondrial DNA contains only 37 genes encoding the two ribosomal RNAs, 22 transfer RNAs and 13 polypeptides [2] . All other proteins, including translation factors and ribosomal proteins, are imported from the cytosol. The mitoribosome is in many ways similar to bacterial ribosomes and several of its translation factors show activity on these [3] . This in line with the fact that the key functional regions involved in decoding and peptide bond formation are largely conserved [4] , which they are most likely to be also on the tertiary structure level. Nevertheless, the overall composition and structure of the mitoribosome differs considerably from its bacterial counterpart, for example, with roughly inverted protein-to-RNA ratio [5] of about 3:1 and a larger total mass [6] . Although evolution has led to a universal genetic code, many examples of deviations exist [7] , [8] . In vertebrate mitochondria, the standard stop codon UGA has been reassigned to encode tryptophan, whereas the two arginine codons AGA and AGG have no cognate tRNAs and have instead been reassigned to stop codons in many organisms [2] . For example, in human mitochondria the CO1 and ND6 genes end with AGA and AGG stop codons, respectively [2] . Interestingly, four different human proteins homologous to the bacterial release factor RF1 have been found [9] : mtRF1, mtRF1a, ICT1 and C12orf65. mtRF1 was identified by bioinformatics and was initially believed to read all four of the mitochondrial stop codons [10] . A new candidate, mtRF1a, was later found and shown to have release activity in vitro on Escherichia coli ribosomes for the UAA and UAG stop codons [11] , [12] . However, no release activity for mtRF1 was observed at any of the mitochondrial stop codons UAA, UAG, AGA and AGG in these bacterial termination assays. Yet, the possibility of mtRF1 being responsible for reading the non-standard stop codons on the mitoribosome cannot be excluded [13] , as it has two insertions in the region reading the first stop codon position [14] , which might confer the ability to read an adenine. These insertions consist of three amino acids (Gly–Leu–Ser) in the stop codon recognition loop and two residues (Arg–Thr) in the short loop preceding the α5 helix. The other two homologues of the bacterial release factors (RFs), ICT1 and C12orf65, are both mitochondrial proteins with critical functions for cell viability and have been proposed to be involved in rescuing stalled ribosomes [9] , [15] , [16] . ICT1 has further been shown to be an integral part of the mitoribosome [9] . However, both proteins lack the codon recognition domain of RF1 and RF2, which is present in mtRF1 and mtRF1a. The termination mechanism in mitochondria thus remains an unsolved problem and it is still unclear whether there are one or two mitochondrial release factors (mtRFs) and whether there actually are two or four stop codons in vertebrate mitochondria. Previous studies have suggested two different hypotheses for the termination at non-standard stop codons, where the first invokes RNA editing [11] and the second a −1 frameshift [17] , both leading to the mtRFs effectively reading a UAG codon. Neither of these hypotheses can be completely verified or disproved without an in vitro vertebrate mitochondrial translation assay, but no such system is available at present. However, computational modelling and molecular dynamics (MD) simulations have been remarkably successful in predicting key features of several steps involved in the translation process [18] , including termination by class-1 RFs [19] , [20] , and may offer a useful strategy for exploring the mitochondrial termination problem. Here we first employ homology modelling based on the structure of RF1 in complex with the bacterial ribosome [14] to derive structural models of mtRF1a and mtRF1. These models are then used to determine codon specificities through extensive MD simulations and free-energy calculations. The results show that neither of the two factors is able to read AGA or AGG. Instead, we present an alternative mechanism by which ICT1 causes termination. Homology modelling Homology models of mtRF1a and mtRF1 were created with automated protocols using the crystal structure of the Thermus thermophilus RF1–ribosome complex [14] as a template, including the stop codon. Sequence alignments of the RF regions close to the stop codon and the ribosomal A-site are shown in Fig. 1 together with the predicted three-dimensional structures. The overall sequence identities for mtRF1a and mtRF1 with RF1 are 47% and 39%, respectively, and the values for the stop codon recognition domain are very similar. mtRF1a has a high sequence identity with bacterial RF1 in the stop codon recognition region ( Fig. 1a ) and could thus be expected to have analogous codon-reading properties. mtRF1, on the other hand, is similar to RF1 around the third stop codon position but is distinctly different near the first and second positions, where the two insertions are present. As mentioned above, mtRF1 has an RT insertion just before the α5 helix and a GLS insertion in the recognition loop ( Fig. 1c ). Because of these insertions, it appears essential to include (the conserved) rRNA bases close to the recognition loop in the template to avoid unrealistic loop conformations. It was further noted that A1913 in the bacterial large subunit helix 69, interacting with RF1, corresponds to a C in the human mitoribosome, and this substitution was also included in the template. 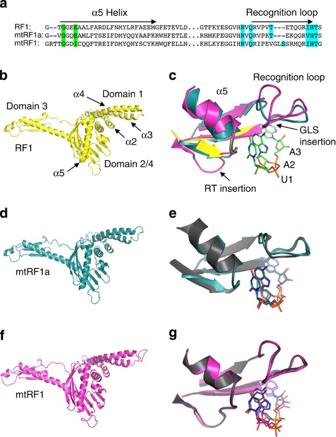Figure 1: Structural comparisons of release factors. (a) Sequence alignments withT. thermophilusRF1 used in the homology modelling of mtRF1a and mtRF1. Residues involved in first position reading are coloured in green (note that these are backbone interactions) and those involved in the second and third position reading are shown in cyan. (b) RF1 crystal structure in the ribosome complex14. (c) Close-up image of the decoding region with the homology models of mtRF1a (cyan) and mtRF1 (magenta) superimposed on the crystal structure of the RF1–ribosome complex (yellow) with the UAA stop codon (shown in stick representation). (d) Overall homology model of mtRF1a. (e) Average structure of mtRF1a (grey) after MD equilibration of the termination complex superimposed on the initial homology model (cyan). (f) Overall homology model of mtRF1. (g) Average structure of mtRF1 (grey) after MD equilibration of the termination complex superimposed on the initial homology model (magenta). Figure 1: Structural comparisons of release factors. ( a ) Sequence alignments with T. thermophilus RF1 used in the homology modelling of mtRF1a and mtRF1. Residues involved in first position reading are coloured in green (note that these are backbone interactions) and those involved in the second and third position reading are shown in cyan. ( b ) RF1 crystal structure in the ribosome complex [14] . ( c ) Close-up image of the decoding region with the homology models of mtRF1a (cyan) and mtRF1 (magenta) superimposed on the crystal structure of the RF1–ribosome complex (yellow) with the UAA stop codon (shown in stick representation). ( d ) Overall homology model of mtRF1a. ( e ) Average structure of mtRF1a (grey) after MD equilibration of the termination complex superimposed on the initial homology model (cyan). ( f ) Overall homology model of mtRF1. ( g ) Average structure of mtRF1 (grey) after MD equilibration of the termination complex superimposed on the initial homology model (magenta). Full size image Modelling of mtRF1 with the included rRNA and the A1913C mutation resulted in a very reasonable structure where mtRF1 makes a hydrogen bond to the cytosine, similar to the interaction between Thr115 in RF1 and A1913 ( Fig. 2 ). Arg193 of the RT insertion is predicted to adopt the position occupied by Arg298 in the so-called switch loop of RF1. Furthermore, in mtRF1 Arg298 corresponds to a glutamine and the switch loop is slightly shifted away, which increases the space for the RT loop to fit without disrupting the positioning of the rRNA. Thr194 of the insertion further stabilizes this conformation of the loop by hydrogen bonding to β5 ( Fig. 2 ). In the recognition loop, the characteristic PxT motif corresponds to PKT in mtRF1a, whereas mtRF1 has a longer loop due to the GLS insertion. Here the loop in mtRF1 is predicted to adopt a conformation so that the inserted Ser169 aligns with the position of Thr186 in RF1 (see below), allowing the serine to bridge between the first and second codon positions of UAA as seen in crystal structures [14] . The homology model of mtRF1 actually shows more favourable interactions with the large subunit than mtRF1a, which has a valine at the position of Thr115 in RF1 and no polar contacts with the A1913C base. 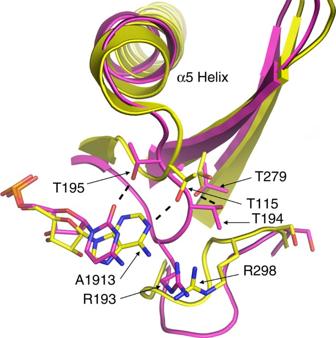Figure 2: Conformation and interactions of the RT loop in the mtRF1 homology model. The mtRF1 homology model (magenta) aligned on the RF1 crystal structure (yellow). The mitochondrial A1913C mutation creates sufficient space for the RT insertion to be able to fit and interact favourably with the ribosome. Figure 2: Conformation and interactions of the RT loop in the mtRF1 homology model. The mtRF1 homology model (magenta) aligned on the RF1 crystal structure (yellow). The mitochondrial A1913C mutation creates sufficient space for the RT insertion to be able to fit and interact favourably with the ribosome. Full size image Despite strong conservation among the three RFs in several regions, the sequence homology deteriorates distinctly upstream of the loop connecting domains 1 and 2, and the entire domain 1 differs considerably. It is clear that its contact regions with both the small and large ribosomal subunits are bound to be different in mtRF1. For example, there appears to be an insertion in the loop connecting helices α3 and α4 that would be likely to collide with rRNA helices 33 and 33a of the bacterial 30S subunit. Notably, these two rRNA helices are deleted in vertebrate mitoribosomes [5] . Similarly, the contact points between domain 1 and the 50S subunit involve sequences at the amino terminus of α3 and carboxy terminus of α4 where the RFs have very low homology. On the bacterial 50S subunit, these contact regions involve rRNA helices 43–44 and 95 to which the linker sequences have been shortened considerably in vertebrate mitoribosomes, which could imply a different positioning of the helices. Hence, shortening of the rRNA in the mitoribosome in regions distant from the decoding centre may well explain why mtRF1 shows no release activity with bacterial ribosomes. To further explore the decoding characteristics of mtRF1a and mtRF1, MD simulations and free-energy calculations were performed with the homology models in the ribosomal A-site [14] , including the A1913C mutation. Here the initial MD simulations also serve as a refinement procedure that allows relaxation of the static models. In particular, it is necessary to evaluate the stability of the two loop insertions in mtRF1. As can be seen from Fig. 1e,g , the predicted structures of both mtRF1a and mtRF1 are remarkably stable during MD simulation with the template UAA codon in the ribosomal A-site and also have favourable backbone characteristics ( Supplementary Fig. S1 ). Energetics of stop codon reading The MD free-energy calculations involve computing the relative binding free energies ( ΔΔG bind ) for the RFs between the cognate RF1 codons UAA and UAG, and the non-cognate codons UGA, AAA and AGA. For comparison, simulations of RF1 and RF2 binding to the bacterial ribosome were also carried out and the cognate-to-cognate UAA to UAG and UAA to UGA mutations for RF1 and RF2, respectively, thus serve as controls of cognate codon recognition. The calculated binding free energies are summarized in Fig. 3a (see also Supplementary Table S1 ), and provide a clear picture of the recognition pattern of the two mitochondrial RFs. As found earlier [20] , the calculated binding free energies for RF1 are very similar to those derived from experimental K M values [21] . Both mtRF1a and mtRF1 are predicted to behave qualitatively the same as RF1, with large discriminations towards both a first-position A and a second-position G. This is evident from both mutations of UAA into AAA and UGA, and the mutation of UGA into AGA. Moreover, the differences in binding affinity between UAA and UGA for mtRF1a and mtRF1 are large (+3.5 and +6.0 kcal mol −1 , respectively) compared with RF2 (−0.6 kcal mol −1 ) for which UGA is cognate. Hence, there is no sign of either mtRF1a or mtRF1 being able to read the first two bases of the non-standard stop codons AGA and AGG. Just as for RF1, both mtRF1a and mtRF1 are found to be insensitive to A/G substitution at the third codon position, in accordance with the conservation of the key RF1 residues Gln181 and Thr194 (ref. 20 ). 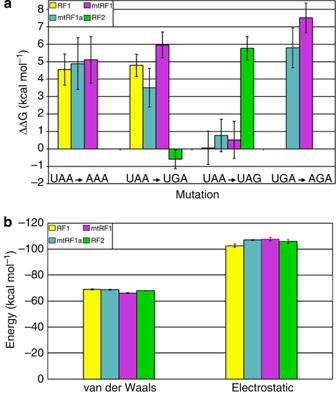Figure 3: Stop codon specificity of mitochondrial and bacterial release factors. (a) Calculated changes in binding free energy (kcal mol−1) for termination complexes with mtRF1a, mtRF1, RF1 and RF2 caused by different stop codon mutations. (b) Average interaction energies between the UAA codon bases and their surrounding environment for RF1 (yellow), mtRF1a (cyan), mtRF1 (magenta) and RF2 (green). Errors are given as the s.e.m. for ten independent simulations. Figure 3: Stop codon specificity of mitochondrial and bacterial release factors. ( a ) Calculated changes in binding free energy (kcal mol −1 ) for termination complexes with mtRF1a, mtRF1, RF1 and RF2 caused by different stop codon mutations. ( b ) Average interaction energies between the UAA codon bases and their surrounding environment for RF1 (yellow), mtRF1a (cyan), mtRF1 (magenta) and RF2 (green). Errors are given as the s.e.m. for ten independent simulations. Full size image The question of whether mtRF1 has the ability to bind any stop codon at all is not addressed by the free-energy calculations in Fig. 3a , as they only yield binding free energies relative to UAA. However, by calculating the average MD interaction energies of the UAA codon for the four ribosome complexes with RF1, mtRF1a, mtRF1 and RF2 as done in earlier work on codon–anticodon recognition [22] , the absolute binding affinities of the four factors for UAA can be compared. This shows that the affinities in the decoding site are expected to be similar for all four release factors ( Fig. 3b ). Hence, although it is still beyond the scope of current simulation methods to predict absolute binding free energies to the entire ribosome, we can conclude that there is no indication of any major affinity differences among the different RFs for the messenger RNA codon. Structural basis of mtRF1a and mtRF1 stop codon specificity Besides yielding very similar interaction energies, the MD simulations with the UAA stop codon also show that the key interactions between the codon and the RFs are largely conserved ( Fig. 4 ). Hence, just as in RF1 and RF2 the N terminus of the α5 helix with its conserved glycines reads the first-position U in both mtRF1a and mtRF1. Further, as noted above, Ser269 in the recognition loop of mtRF1 replaces the role of Thr186 in the RF1 PxT motif and recognizes both the first-position U and second-position A ( Fig. 4c ), which would not have been expected from the sequence alignment alone. The positioning of Ser269 in mtRF1 is consistently predicted both by the homology model and MD simulations. 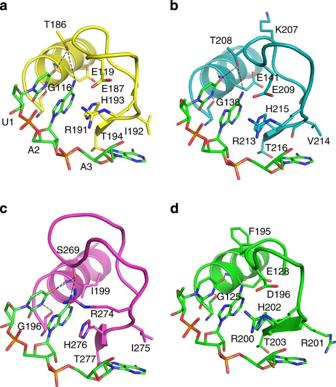Figure 4: Comparison of UAA reading by different release factors. (a–d) Average structures from MD simulations of RF1 (yellow), mtRF1a (cyan), mtRF1 (magenta) and RF2 (green) with key residues in stick representation and hydrogen bonds shown as dashed lines. The hydrogen bond network in the reading of UAA is similar for RF1, mtRF1a and mtRF1 in all three stop codon positions. Ser269 in mtRF1 interacts with U1 and A2 in a similar fashion as Thr206 in mtRF1a and Thr186 in RF1. Figure 4: Comparison of UAA reading by different release factors. ( a–d ) Average structures from MD simulations of RF1 (yellow), mtRF1a (cyan), mtRF1 (magenta) and RF2 (green) with key residues in stick representation and hydrogen bonds shown as dashed lines. The hydrogen bond network in the reading of UAA is similar for RF1, mtRF1a and mtRF1 in all three stop codon positions. Ser269 in mtRF1 interacts with U1 and A2 in a similar fashion as Thr206 in mtRF1a and Thr186 in RF1. Full size image To further compare the structural features of stop codon reading, and possibly identify putative hotspots for AGA and AGG reading, average MD structures for mtRF1a and mtRF1 were analysed. 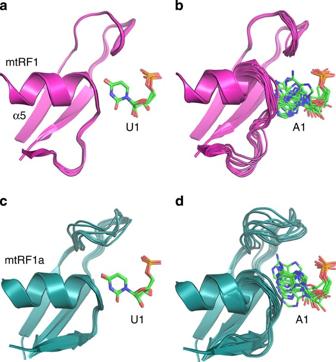Figure 5: Codon reading at the first position. (a) Average structures of ten independent MD simulations of mtRF1 (magenta) in complex with UAA (U1 in sticks), showing good structural convergence. (b) Average structures from the corresponding simulations with AAA show A1 shifted away from the tip of α5, with a less well-defined conformation. (c,d) Average structures from corresponding MD simulations of mtRF1a with the UAA and AAA codons, respectively. Figure 5 shows the average structures from ten independent simulations of mtRF1a and mtRF1 with the UAA and AAA codons. With a first-position A, there is no unique stable conformation of the nucleotide, which is shifted away from the α5 helix disrupting the preceding loop structure for both of the mtRFs. In contrast, with a first-position U, the structures are remarkably stable ( Fig. 5 ). Hence, it is evident for both mtRF1a and mtRF1 that there is too limited space for accommodating a purine at the first stop codon position owing to the location of the α5 helix. In particular, none of the mtRF1 insertion residues show any sign of favourable interactions with a first-position A, in contrast to the UAA codon, which shows the same strong hydrogen bonds with the α5 helix and the recognition loop that have previously been identified [14] , [20] . Figure 5: Codon reading at the first position. ( a ) Average structures of ten independent MD simulations of mtRF1 (magenta) in complex with UAA (U1 in sticks), showing good structural convergence. ( b ) Average structures from the corresponding simulations with AAA show A1 shifted away from the tip of α5, with a less well-defined conformation. ( c , d ) Average structures from corresponding MD simulations of mtRF1a with the UAA and AAA codons, respectively. Full size image The key residue enabling reading of a second-position G in RF2 is Glu128, the position of which is controlled by specific interaction network of mostly charged residues [20] , [23] . Although this residue is also a glutamate in RF1 (Glu119) and mtRF1a (Glu141), its interaction network is different in these RFs, prohibiting an efficient interaction with G2 as described earlier [20] . However, in mtRF1, the residue at this position is Ile199 and the entire cavity that would accommodate a second-position G is mostly hydrophobic. Hence, it is clear that Ile199 cannot contribute to a higher specificity for accommodating a G in the second position. This is illustrated in Fig. 6 where the average MD structures of RF2 and mtRF1 with the UGA codon are shown together with average G2 interaction energies with the binding site. mtRF1 shows no stabilization of a second-position G in contrast to RF2 where Glu128 is the key specificity element. 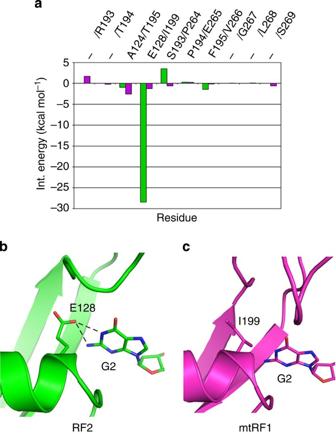Figure 6: The second-position binding pocket in mtRF1 cannot accommodate a G. (a) Average interaction energies between G2 and the surrounding amino acids from MD simulations with the UGA codon show no stabilization of the second position G in mtRF1, in contrast to the case with bacterial RF2. Residue numbers are given in the format RF2/mtRF1, and green and magenta bars denote RF2 and mtRF1 energies, respectively. (b,c) Average structures of RF2 (green) and mtRF1 (magenta) zoomed in on the second stop codon position. Ile199 is unable to form the hydrogen bonds with G2 seen in the RF2 UGA complex. Figure 6: The second-position binding pocket in mtRF1 cannot accommodate a G. ( a ) Average interaction energies between G2 and the surrounding amino acids from MD simulations with the UGA codon show no stabilization of the second position G in mtRF1, in contrast to the case with bacterial RF2. Residue numbers are given in the format RF2/mtRF1, and green and magenta bars denote RF2 and mtRF1 energies, respectively. ( b , c ) Average structures of RF2 (green) and mtRF1 (magenta) zoomed in on the second stop codon position. Ile199 is unable to form the hydrogen bonds with G2 seen in the RF2 UGA complex. Full size image Apart from the insertion residues in the recognition loop, mtRF1 shows a difference in the positioning of Arg274 compared with the corresponding Arg residue in RF1, RF2 and mtRF1a. This appears to be caused by the absence of the negatively charged residue found in the other RFs (Glu187 in RF1, Asp196 in RF2 and Glu209 in mtRF1a), which in mtRF1 allows Arg274 to form strong interactions with the mRNA backbone of the first stop codon position and the second position base ( Supplementary Fig. S2 ). In addition, Arg274 makes hydrogen bonds with both Ser269 and His276, as well as with the sugar backbone of the P-site mRNA via a bridging water molecule. This extensive hydrogen bond network of Arg274 thus contributes to stabilization of the considerably larger recognition loop in mtRF1. An alternative mechanism for AGA and AGG termination To investigate the reported hydrolysis induced by ICT1 at the non-standard stop codons [9] , a homology model of ICT1 was constructed based on the structure of the bacterial homologue YaeJ. YaeJ is a rescue factor for stalled ribosomes and its ribosome complex was solved with a short mRNA ending in the P-site, as would be the case for stalled ribosomes with an empty A-site [24] . In this structure, the C-terminal tail of YaeJ is positioned in the mRNA channel, where it is able to detect the missing A-site codon. Moreover, YaeJ has been shown to rescue ribosomes stalled due to rare AGG codon clusters [25] . Interestingly, the path of the C-terminal tail of YaeJ observed in the crystal structure [24] would not be possible with a codon in the A-site, as the tail would clash with the mRNA. Moreover, the observed peptidyl-tRNA hydrolysis caused by ICT1 with several codons (including AGA and AGG) [9] therefore suggests that the crystal structure path of YaeJ [24] is not compatible with ICT1 binding with an A-site codon present. However, two alternative paths of YaeJ can, in fact, be identified and Fig. 7a shows these conformations together with the crystal structure of YaeJ, aligned to a ribosome with A-site mRNA present [26] . 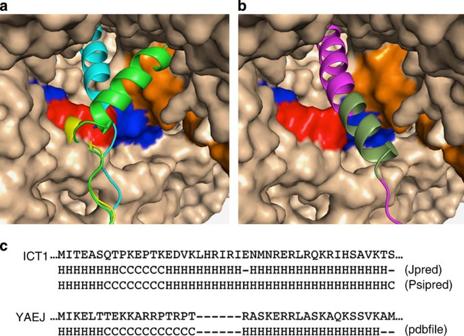Figure 7: A model for mitochondrial termination with ICT1. (a) Two possible paths for YaeJ (green and cyan) with mRNA (blue) present in the mRNA channel. The A-site codon in highlighted in red and the P-site tRNA is shown in orange. The yellow structure corresponds to the known path of YaeJ on a ribosome without an A-site codon and with an empty mRNA channel. (b) Homology model of ICT1 (magenta) positioned in one of the possible paths. The insertion in ICT1 and four additional amino acids were modelled as an extension (dark green) of the α-helix according to the secondary structure prediction. (c) Alignment and secondary structure prediction of the C-terminal end or ICT1 and YaeJ. Figure 7: A model for mitochondrial termination with ICT1. ( a ) Two possible paths for YaeJ (green and cyan) with mRNA (blue) present in the mRNA channel. The A-site codon in highlighted in red and the P-site tRNA is shown in orange. The yellow structure corresponds to the known path of YaeJ on a ribosome without an A-site codon and with an empty mRNA channel. ( b ) Homology model of ICT1 (magenta) positioned in one of the possible paths. The insertion in ICT1 and four additional amino acids were modelled as an extension (dark green) of the α-helix according to the secondary structure prediction. ( c ) Alignment and secondary structure prediction of the C-terminal end or ICT1 and YaeJ. Full size image Sequence alignment of human ICT1 and E. coli YaeJ also reveals an insertion of six residues in ICT1 preceding the α-helix at the end of YaeJ. This insertion is consistently assigned by secondary structure prediction tools [27] , [28] to be a part of the C-terminal helix ( Fig. 7c ). The homology model of ICT1 was created based on one of the alternative paths of YaeJ as template. The insertion predicted to be part of the helix is then positioned close to the A-site codon ( Fig. 7b ). Similar to YaeJ, this part of the helix has several positively charged residues that could interact with the phosphate backbone of the mitoribosome and possibly the mRNA phosphates, thereby providing a termination mechanism for ribosomes stalled at the AGA and AGG codons. The conclusion from our extensive MD free-energy calculations on the homology models of mtRF1a and mtRF1 is that neither of these RFs is able to cause termination at the non-standard stop codons. Instead, we find that both mtRF1a and mtRF1 behave very much like the bacterial RF1, both with regard to codon specificity and interactions of key residues involved in codon binding [20] . The ability to read a first-position purine, as would be required for the AGA and AGG codons, is essentially prevented by the position of the α5 helix, which is highly unlikely to differ between the mtRFs and RF1. Even though the bacterial and the mitochondrial ribosomes are bound to be rather different overall, the fact that the decoding region of the mitochondrial 9S and the bacterial 16S RNA are conserved in secondary structure [4] , [29] strongly suggests that this also pertains on the local three-dimensional structure. This is also supported by the strong sequence conservation between RF1 and mtRF1a in the decoding region, which, together with the fact that the experimentally observed specificity of mtRF1a on bacterial ribosomes [11] , [12] , is reproduced here, strengthens the reliability of our derived homology models. One of the two main hypotheses regarding termination at non-standard stop codons suggested a mechanism based on a −1 frameshift [17] . This would in human mitochondria result in the standard UAG stop codon, as both CO1 and ND6 has a U preceding AGA and AGG, respectively. This experimental evidence for this theory relies entirely on the capability of RelE to only cut the mRNA between the second and third position, which can, however, be questioned, as RelE has shown activity at different positions and codons in vivo [30] . Furthermore, it has been pointed out that human mitochondria are not the only vertebrate ones using non-standard stop codons [13] . Bioinformatics investigations have, in fact, shown that a U preceding AGA and AGG is rare [31] and Supplementary Table S2 shows a few examples of vertebrates using non-standard stop codons, where most of the preceding codons end with an A. The second hypothesis suggests that mtRF1 is the RF causing termination on AGA and AGG. This was mainly based on the ability of a hybrid RF1, which was mutated to resemble mtRF1, to show a rather weak hydrolysis activity at the AAG (and UAA) codon [13] . However, its activity on AGA and AGG was barely above the background with no codon. It would thus seem that the hybrid RF1 has lost both activity and specificity by the mutations introduced, rather than obtaining a possible specificity for an A in the first position. Furthermore, it is clear that there are correlated mutations across the chimeric boundaries used in ref. 13 . For example, the α5 RT insertion is correlated with mutations in the switch loop (see above) in addition to the A1913C rRNA mutation, which explains why the hybrid that only included the RT-insertion region from mtRF1 was completely inactive [13] . As our calculations show no indication of mtRF1a or mtRF1 acting on the non-standard stop codons, this raises the key question whether there is any other possible mechanism for the termination at AGA and AGG. Here the two other members of the mitochondrial RF family, ICT1 and C12orf65, are of considerable interest, as they have been shown to be vital for mitochondrial translation. In fact, the only member of the mtRF family that has shown any in vitro activity on AGA and AGG is ICT1 (ref. 9 ). A mechanism where the mitoribosome becomes stalled at AGA or AGG, which lack cognate tRNAs, and then rescued by ICT1 would provide a possible explanation for the existence of non-standard stop codons. The homology model of ICT1 presented here reveals an extension of the α-helix, which in the YaeJ–ribosome complex [24] is located at the A-site codon position. This helical structure could potentially assist in sensing a codon for which there is no tRNA and cause termination. Our calculated energetics show that mtRF1a and mtRF1 have overlapping specificities for the UAA and UAG stop codons, comparable to the overlapping specificity for UAA by RF1 and RF2 in bacteria. This could be one reason for the limited effect on protein levels reported on mtRF1a depletion [12] . It is also a distinct possibility that mtRF1 is, in fact, the major release factor in vertebrate mitochondria, as mtRF1 has apparently not been tested in knockdown experiments. In this respect, measurements of release activity on bacterial ribosomes [11] , [12] may be less relevant for the activity on the mitoribosome. It should also be mentioned that earlier homology modelling suggested that mtRF1 cannot read any codon but recognizes ribosomes with an empty A-site [32] . However, the mtRF1 homology model was in that case based on bacterial RF structures with no rRNA or mRNA included [32] , which may drastically affect the conformational space accessible to the protein. Structural relaxation by MD simulations and free-energy calculations further provide critical tests of the stability and energetics associated with homology models and are essential for drawing conclusions regarding binding properties. What speaks in favour of mtRF1 being the major release factor is the fact that the emergence of mtRF1 in vertebrates appears to be correlated with major changes in the mt-rRNA. That is, the consistent shortening of the mt-rRNA in vertebrates may have required concomitant adaptation of a release factor to be effective on these mitoribosomes. mtRF1 could thus be a factor that has specifically co-evolved with the vertebrate mitoribosome to adapt to its new rRNA structure. Another observation that may support a key role for mtRF1 is that its discrimination against UGA (which codes for Trp in vertebrate mitochondria) is predicted here to be significantly stronger than that of mtRF1a. As noted above, the key mutation to a hydrophobic residue (Ile199) near the second codon position strongly prevents UGA reading, suggesting that mtRF1 is evolved for the recoding of this codon in mitochondria. Homology modelling Homology models of mtRF1a and mtRF1 were created using Prime 2.1 (Schrödinger, LLC, New York, NY, 2007) and Modeller (Version 9.10) [33] with the bacterial RF1–ribosome complex [14] as template, including nearby rRNA, the stop codon and the A1913C mutation. The homology model of ICT1 was created with Prime 2.1 and the crystal structure of YaeJ–ribosome complex [24] as template. The alignment was further compared with the solution structure of the Mus musculus ICT1 (ref. 34 ) to get the correct secondary structure alignment. The helix close to the C-terminal end (missing in ref. 34 ) was modelled as predicted by PSIPRED [28] ( Fig. 7 ). The model was minimized in MacroModel 9.5 (Schrödinger, LLC) using the OPLS-AA force field [35] . Molecular dynamics and free-energy simulations Relative binding free energies ( ΔΔG bind ) between different termination complexes were calculated using the free-energy perturbation (FEP) technique (see, for example, Brandsdal et al. [36] ) and a standard thermodynamic cycle [20] . Initial coordinates for the MD and FEP calculations were taken from the crystal structure of RF1 and RF2 bound to the 70S ribosome [14] , [23] and the corresponding homology models of mtRF1 and mtRF1a. For the mtRF1a and mtRF1 structures, A1913 of the 70S ribosome was changed to a C in accordance with the human mitoribosome sequence. The RF histidine residue between the second and third codon position was treated as neutral and protonated at ND1 (as there is an arginine residue close to NE2), and magnesium ion positions were selected from previous calculations [20] . To evaluate the changes in binding free energy, a set of different mRNA codon transformations (mutations) were carried out during MD simulations with and without the relevant release factor bound to the solvated ribosome–mRNA complex. The MD/FEP calculations were carried out with spherical systems (40 Å in diameter) centred on the nucleotide base that was transformed (see Fig. 3 for the different transformations). All MD simulations were carried out with the Q programme [37] using the Charmm22 force field [38] , [39] . The simulations were done at 300 K after stepwise heating of the system from 1 K. Water molecules close to the sphere boundary were subjected to radial and polarization restraints according the SCAAS model [37] , [40] . The MD simulations were carried out with a time step of 1 fs, and solvent bonds and angles were treated with the SHAKE algorithm [41] . Non-bonded interactions were treated with a 10-Å direct cutoff, and long-range electrostatic interactions beyond this cutoff were treated with the local reaction field method [42] . No cutoffs were applied to the transformed bases, and charged groups close to the sphere boundary were neutralized as described elsewhere [43] . Ten independent FEP simulations of each system were performed using different initial conditions. All FEP calculations were carried out using 51 windows ( λ -points) interspaced for optimal efficiency with small λ -steps (0.0008) near the end points, with 200 ps of simulation time for each window [36] , resulting in a total data collection time of 100 ns after equilibration and heating. For all first-position calculations transforming U into A, the dual topology method was used, owing to the larger changes involved when transforming a pyrimidine into a purine, whereas the single topology method was used for A-to-G mutations. How to cite this article: Lind, C. et al. Codon-reading specificities of mitochondrial release factors and translation termination at non-standard stop codons. Nat. Commun. 4:2940 doi: 10.1038/ncomms3940 (2013).